Propagation of an Earth-directed coronal mass ejection in three dimensions Solar coronal mass ejections (CMEs) are the most significant drivers of adverse space weather on Earth, but the physics governing their propagation through the heliosphere is not well understood. Although stereoscopic imaging of CMEs with NASA's Solar Terrestrial Relations Observatory (STEREO) has provided some insight into their three-dimensional (3D) propagation, the mechanisms governing their evolution remain unclear because of difficulties in reconstructing their true 3D structure. In this paper, we use a new elliptical tie-pointing technique to reconstruct a full CME front in 3D, enabling us to quantify its deflected trajectory from high latitudes along the ecliptic, and measure its increasing angular width and propagation from 2 to 46 ( ∼ 0.2 AU). Beyond 7 , we show that its motion is determined by an aerodynamic drag in the solar wind and, using our reconstruction as input for a 3D magnetohydrodynamic simulation, we determine an accurate arrival time at the Lagrangian L1 point near Earth. Coronal mass ejections (CMEs) are spectacular eruptions of plasma and magnetic field from the surface of the Sun into the heliosphere. Travelling at speeds of up to 2,500 km s −1 and with masses of up to 10 16 g, they are recognized as drivers of geomagnetic disturbances and adverse space weather on Earth and on other planets in the solar system [1] , [2] . Affecting our magnetosphere with average magnetic field strengths of 13 nT and energies of ∼ 10 25 J, they can cause telecommunication and Global Positioning System (GPS) errors, power grid failures and increased radiation risks to astronauts [3] . It is therefore important to understand the forces that determine their evolution, in order to better forecast their arrival time and impact on Earth and throughout the heliosphere. Identifying the specific processes that trigger the eruption of CMEs is the subject of much debate, and many different models exist to explain these [4] , [5] , [6] . One common feature is that magnetic reconnection is responsible for the destabilization of magnetic flux ropes on the Sun, which then erupt through the corona into the solar wind to form CMEs [7] . In the low solar atmosphere, it is postulated that high-latitude CMEs undergo deflection as they are often observed at different position angles than their associated source region locations [8] . It has been suggested that field lines from polar coronal holes may guide high-latitude CMEs towards the equator [9] , or that the initial magnetic polarity of a flux rope relative to the background magnetic field influences its trajectory [10] , [11] . During this early phase, CMEs are observed to expand outwards from their launch site, although plane-of-sky measurements of their increasing sizes and angular widths are ambiguous in this regard [12] . This expansion has been modelled as being due to a pressure gradient between the flux rope and the background solar wind [13] , [14] . At larger distances in their propagation, CMEs are expected to interact with the solar wind and the interplanetary magnetic field. Studies that compare in situ CME velocity measurements with initial eruption speeds through the corona show that slow CMEs are accelerated towards the speed of the solar wind, and fast CMEs decelerated [15] , [16] . It has been suggested that this is due to the effects of drag on the CME in the solar wind [17] , [18] . However, the quantification of drag, along with that of both CME expansion and non-radial motion, is currently lacking, primarily because of the limits of observations from single fixed viewpoints with restricted fields of view. The projected two-dimensional nature of these images introduces uncertainties in kinematical and morphological analyses, and therefore the true three-dimensional (3D) geometry and dynamics of CMEs have been difficult to resolve. Efforts were made to infer 3D structure from two-dimensional images recorded by the large angle spectrometric coronagraph on board the Solar and Heliospheric Observatory, situated at the first Lagrangian point (L1), at which its orbital motion around the Sun is synchronous with that of the Earth's. These efforts were based on either a preassumed geometry of the CME [19] , [20] , [21] or a comparison of observations with in situ and on-disk data [22] , [23] . Of note is the polarization technique used to reconstruct the 3D geometry of CMEs in large angle spectrometric coronagraph data [24] , although this is only valid for heights of up to 5 (1 ). Recently, new methods to track CMEs in 3D have been developed for the Solar Terrestrial Relations Observatory (STEREO) mission [25] . Launched by NASA in 2006, STEREO consists of two near-identical spacecrafts in heliocentric orbits ahead and behind the Earth, which drift away from the Sun–Earth line at a rate of ± 22° per year. This provides a unique twin perspective of the Sun and inner heliosphere, and enables the implementation of a variety of methods for studying CMEs in 3D [26] . Many of these techniques are applied within the context of an epipolar geometry [27] . One such technique consists of tie-pointing lines of sight across epipolar planes, and is best for resolving a single feature such as a coronal loop on-disk [28] . Under the assumption that the same feature may be tracked in coronagraph images, many CME studies have also used tie-pointing techniques with the COR1 and COR2 coronagraphs of the Sun-Earth Connection Coronal and Heliospheric Investigation (SECCHI [29] ) aboard STEREO [30] , [31] , [32] . The additional use of SECCHI's Heliospheric Imagers (HI1/2) allows a study of CMEs out to distances of 1 astronomical unit (1 AU=149.6×10 6 km); however, a 3D analysis can only be carried out if the CME propagates along a trajectory between the two spacecrafts so that it is observed by both HI instruments. Otherwise, assumptions of its trajectory have to be inferred from either its association with a source region on-disk [33] or its trajectory through the COR data [15] , or derived by assuming a constant velocity through the HI fields of view [34] . Triangulation of CME features using time-stacked intensity slices at a fixed latitude, named 'J-maps' because of the characteristic propagation signature of a CME, has also been developed [35] , [36] . This technique is hindered by the same limitation of standard tie-pointing techniques, namely, that the curvature of the feature is not considered, and the intersection of sight lines may not occur on the surface of the observed feature. Alternatively, forward modelling of a 3D flux rope based on a graduated cylinder model may be applied to STEREO observations [37] . Some of the parameters governing the model shape and orientation may be changed by the user to best fit the twin observations simultaneously, although the assumed flux rope geometry is not always appropriate. We have developed a new 3D triangulation technique that overcomes the limitations of previous methods by considering the curvature of the CME front in the data. This functions as a necessary third constraint on the reconstruction of the CME front from the combined observations of the twin STEREO spacecraft. Applying this to every image in the sequence enables us to investigate the changing dynamics and morphology of the CME as it propagates from the Sun into interplanetary space. CME observation On 12 December 2008, an erupting prominence was observed by STEREO while the spacecraft was in near quadrature at 86.7° separation ( Fig. 1a ). The eruption were visible at 50–55° north from 03:00 UT in SECCHI/Extreme Ultraviolet Imager (EUVI) images, obtained in the 304 Å passband, in the northeast from the perspective of STEREO-(A)head and off the northwest limb from STEREO-(B)ehind. The prominence is considered to be the inner material of the CME, which was first observed in COR1-B at 05:35 UT ( Fig. 1b ). For our analysis, we use the two coronagraphs (COR1/2) and the inner HI1 ( Fig. 1c ). We characterize the propagation of the CME across the plane of sky by fitting an ellipse to the front of the CME in each image [38] ( Supplementary Movie 1 ). This ellipse fitting is applied to the leading edges of the CME but equal weight is given to the CME flank edges as they enter the field of view of each instrument. The 3D reconstruction is then performed using a method of elliptical tie pointing within epipolar planes containing the two STEREO spacecraft, illustrated in Figure 2 (see Methods section). 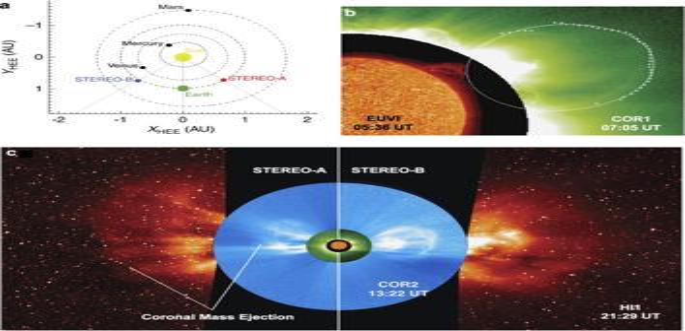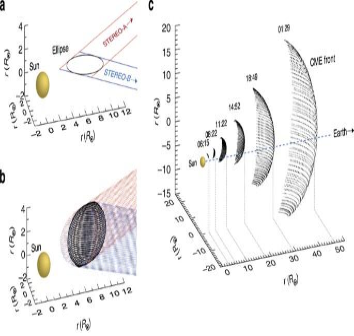Figure 2: Epipolar geometry used to constrain the reconstruction of the CME front. The reconstruction is performed using an elliptical tie-pointing technique within epipolar planes containing the two STEREO spacecraft27. For example, one of any number of planes will intersect the ellipse characterization of the CME at two points in each image from STEREO-A and B. (a) Illustrates how the resulting four sight lines intersect in 3D space to define a quadrilateral that constrains the CME front in that plane56,57. Inscribing an ellipse within the quadrilateral such that it is tangent to each sight line58,59provides a slice through the CME that matches the observations from each spacecraft. (b) Illustrates how a full reconstruction is achieved by stacking multiple ellipses from the epipolar slices. As the positions and curvatures of these inscribed ellipses are constrained by the characterized curvature of the CME fronts in the stereoscopic image pair, the modelled CME front is considered to be an optimum reconstruction of the true CME front. (c) Illustrates how this is repeated for every frame of the eruption to build the reconstruction as a function of time and view the changes to the CME front as it propagates in 3D. Although the ellipse characterization applies to both the leading edges and, when observable, the flanks of the CME, only the outermost part of the reconstructed front is shown here for clarity, and illustrated inSupplementary Movie 2. Figure 1: Composite of STEREO-A and B images from the SECCHI instruments of the CME of 12 December 2008. (a) Indicates the STEREO spacecraft locations, separated by an angle of 86.7° at the time of the event. (b) Shows the prominence eruption observed in EUVI-B off the northwest limb from approximately 03:00 UT, which is considered to be the inner material of the CME. The multiscale edge detection and corresponding ellipse characterization are overplotted in COR1. (c) Shows that the CME is Earth-directed, being observed off the east limb in STEREO-A and off the west limb in STEREO-B. Figure 1: Composite of STEREO-A and B images from the SECCHI instruments of the CME of 12 December 2008. ( a ) Indicates the STEREO spacecraft locations, separated by an angle of 86.7° at the time of the event. ( b ) Shows the prominence eruption observed in EUVI-B off the northwest limb from approximately 03:00 UT, which is considered to be the inner material of the CME. The multiscale edge detection and corresponding ellipse characterization are overplotted in COR1. ( c ) Shows that the CME is Earth-directed, being observed off the east limb in STEREO-A and off the west limb in STEREO-B. Full size image Figure 2: Epipolar geometry used to constrain the reconstruction of the CME front. The reconstruction is performed using an elliptical tie-pointing technique within epipolar planes containing the two STEREO spacecraft [27] . For example, one of any number of planes will intersect the ellipse characterization of the CME at two points in each image from STEREO-A and B. ( a ) Illustrates how the resulting four sight lines intersect in 3D space to define a quadrilateral that constrains the CME front in that plane [56] , [57] . Inscribing an ellipse within the quadrilateral such that it is tangent to each sight line [58] , [59] provides a slice through the CME that matches the observations from each spacecraft. ( b ) Illustrates how a full reconstruction is achieved by stacking multiple ellipses from the epipolar slices. As the positions and curvatures of these inscribed ellipses are constrained by the characterized curvature of the CME fronts in the stereoscopic image pair, the modelled CME front is considered to be an optimum reconstruction of the true CME front. ( c ) Illustrates how this is repeated for every frame of the eruption to build the reconstruction as a function of time and view the changes to the CME front as it propagates in 3D. Although the ellipse characterization applies to both the leading edges and, when observable, the flanks of the CME, only the outermost part of the reconstructed front is shown here for clarity, and illustrated in Supplementary Movie 2 . Full size image Non-radial CME motion It is immediately evident from the reconstruction in Figure 2c (and Supplementary Movie 2 ) that the CME propagates non-radially away from the Sun. The CME flanks change from an initial latitude span of 16–46° to finally span approximately ± 30° of the ecliptic ( Fig. 3b ). The mean declination, θ , of the CME is well fitted by a power law of the form as a result of this non-radial propagation. Tie pointing the prominence apex and fitting a power law to its declination angle result in , implying a source latitude of in agreement with EUVI observations. Previous statistics on CME position angles have shown that, during solar minimum, they tend to be offset closer to the equator as compared with those of the associated prominence eruption [39] . The non-radial motion we quantify here may be evidence of the drawn-out magnetic dipole field of the Sun, an effect predicted at solar minimum because of the influence of solar wind pressure [40] , [41] . Other possible influences include changes to the internal current of the magnetic flux rope [11] , or the orientation of the magnetic flux rope with respect to the background field [10] , whereby magnetic pressure can function asymmetrically to deflect the flux rope poleward or equatorward depending on the field configurations. 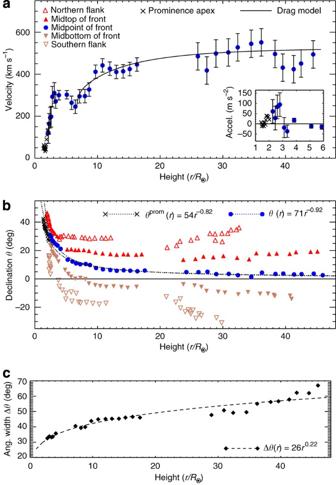Figure 3: Kinematics and morphology of the 3D reconstruction of the CME front of 12 December 2008. (a) Shows the velocity of the middle of the CME front with the corresponding drag model and, inset, the early acceleration peak. Measurement uncertainties are indicated by one standard deviation error bars. (b) Shows the declinations from the ecliptic (0°) of an angular spread across the front between the CME flanks, with a power-law fit indicative of non-radial propagation. It should be noted that the positions of the flanks are subject to large scatter: as the CME enters each field of view, the location of a tangent to its flanks is prone to moving back along the reconstruction in cases in which the epipolar slices completely constrain the flanks. Hence the 'Midtop/Midbottom of Front' measurements better convey the southward-dominated expansion. (c) Shows the angular width of the CME with a power-law expansion. For each instrument, the first three points of angular width measurement were removed as the CME was still predominantly obscured by each instrument's occulter. Figure 3: Kinematics and morphology of the 3D reconstruction of the CME front of 12 December 2008. ( a ) Shows the velocity of the middle of the CME front with the corresponding drag model and, inset, the early acceleration peak. Measurement uncertainties are indicated by one standard deviation error bars. ( b ) Shows the declinations from the ecliptic (0°) of an angular spread across the front between the CME flanks, with a power-law fit indicative of non-radial propagation. It should be noted that the positions of the flanks are subject to large scatter: as the CME enters each field of view, the location of a tangent to its flanks is prone to moving back along the reconstruction in cases in which the epipolar slices completely constrain the flanks. Hence the 'Midtop/Midbottom of Front' measurements better convey the southward-dominated expansion. ( c ) Shows the angular width of the CME with a power-law expansion. For each instrument, the first three points of angular width measurement were removed as the CME was still predominantly obscured by each instrument's occulter. Full size image CME angular width expansion Over the height range of 2–46 , the CME angular width (Δ θ = θ max − θ min ) increases from ∼ 30° to ∼ 60° with a power law of the form ( Fig. 3c ). This angular expansion is evidence of an initial overpressure of the CME relative to the surrounding corona (coincident with its early acceleration inset in Fig. 3a ). The expansion then tends to a constant during the later drag phase of CME propagation, as it expands to maintain pressure balance with heliocentric distance. It is theorized that the expansion may be attributed to two types of kinematic evolution, namely, spherical expansion due to simple convection with the ambient solar wind in a diverging geometry, and expansion due to a pressure gradient between the flux rope and solar wind [13] . It is also noted that the southern portions of the CME manifest the bulk of this expansion below the ecliptic (best observed by comparing the relatively constant 'Midtop of Front' measurements with the more consistently decreasing 'Midbottom of Front' measurements in Fig. 3b ). Inspection of a Wang-Sheeley-Arge solar wind model run [42] reveals higher speed solar wind flows ( ∼ 650 km s −1 ) emanating from open-field regions at high/low latitudes (approximately 30° north/south of the solar equator). Once the initial prominence/CME eruption occurs and is deflected into a non-radial trajectory, it undergoes asymmetric expansion in the solar wind. It is prevented from expanding upwards into the open-field high-speed stream at higher latitudes, and the high internal pressure of the CME relative to the slower solar wind near the ecliptic accounts for its expansion predominantly to the south. In addition, the northern portions of the CME attain greater distances from the Sun than the southern portions as a result of this propagation in varying solar wind speeds, an effect predicted to occur in previous hydrodynamic models [14] . CME drag in the inner heliosphere Investigating the midpoint kinematics of the CME front, we find that the velocity profile increases from approximately 100 to 300 km s −1 over the first 2–5 , before rising more gradually to a scatter between 400 and 550 km s −1 as it propagates outwards ( Fig. 3a ). The acceleration peaks at approximately 100 m s −2 at a height of ∼ 3 , then decreases to scatter about zero. This early phase is generally attributed to the Lorentz force whereby the dominant outward magnetic pressure overcomes the internal and/or external magnetic field tension. The subsequent increase in velocity, at heights above ∼ 7 for this event, is predicted by theory to result from the effects of drag [17] , as the CME is influenced by solar wind flows of ∼ 550 km s −1 emanating from latitudes ≳ ± 5° of the ecliptic (again from inspection of the Wang-Sheeley-Arge model). At large distances from the Sun, during this postulated drag-dominated epoch of CME propagation, the equation of motion can be cast in the following form: This describes a CME of velocity v cme , mass M cme and cross-sectional area A cme propagating through a solar wind flow of velocity v sw and density ρ sw . The drag coefficient C D is found to be of the order of unity for typical CME geometries [18] , whereas the density and area are expected to vary as power-law functions of distance r . Thus, we parameterize the density and geometric variation of the CME and solar wind using a power law [43] to obtain where γ describes the drag regime, which can be either viscous ( γ =1) or aerodynamic ( γ =2), and α and β are constants primarily related to the cross-sectional area of the CME and the density ratio of the solar wind flow to the CME ( ρ sw / ρ cme ). The solar wind velocity is estimated from an empirical model [44] . We determine a theoretical estimate of the CME velocity as a function of distance by numerically integrating Equation (2) using a fourth order Runge–Kutta scheme and fitting the result to the observed velocities from ∼ 7 to 46 . The initial CME height, CME velocity, asymptotic solar wind speed and α , β and γ are obtained from a bootstrapping procedure that provides a final best fit to the observations and confidence intervals of the parameters (see Methods section). Best-fit values for α and β were found to be ( )×10 −5 and , which agree with values found in previous modelling work [44] . The best-fit value for the exponent of the velocity difference between CME and the solar wind, γ , was found to be , which is clear evidence that aerodynamic drag ( γ =2) functions during the propagation of the CME in interplanetary space. The drag model provides an asymptotic CME velocity of km s −1 when extrapolated to 1 AU, which predicts the CME to arrive ∼ 1 day before the Advanced Composition Explorer (ACE) or WIND spacecraft detects it at the L1 point. We investigate this discrepancy by using our 3D reconstruction to simulate the continued propagation of the CME from the Alfvén radius ( ∼ 21.5 ) to Earth using the ENLIL with Cone Model [21] at NASA's Community Coordinated Modeling Center. ENLIL is a time-dependent 3D magnetohydrodynamic code that models CME propagation through interplanetary space. We use the height, velocity and width from our 3D reconstruction as initial conditions for the simulation, and find that the CME is actually slowed to ∼ 342 km s −1 at 1 AU. This is a result of its interaction with an upstream, slow-speed, solar wind flow at distances beyond 50 . This CME velocity is consistent with in situ measurements of solar wind speed ( ∼ 330 km s −1 ) from the ACE and WIND spacecraft at L1. Tracking the peak density of the CME front from the ENLIL simulation gives an arrival time at L1 of ∼ 08:09 UT on 16 December 2008. Accounting for the offset in CME front heights between our 3D reconstruction and ENLIL simulation at distances of 21.5 gives an arrival time in the range of 08:09–13:20 UT on 16 December 2008. This prediction interval agrees well with the earliest derived arrival times of the CME front plasma pileup ahead of the magnetic cloud flux rope from the in situ data of both ACE and WIND ( Fig. 4 ) before its subsequent impact on Earth [34] , [36] . 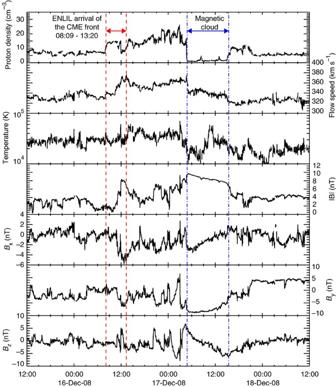Figure 4:In situsolar wind plasma and magnetic field measurements from the WIND spacecraft. From top to bottom, the panels show proton density, bulk flow speed, proton temperature and magnetic field strength and components. The red dashed lines indicate the predicted window of CME arrival time from our ENLIL with Cone Model run (08:09–13:20 UT on 16 December 2008). We observed a magnetic cloud flux rope signature behind the front, highlighted by the blue dash-dotted lines. Figure 4: In situ solar wind plasma and magnetic field measurements from the WIND spacecraft. From top to bottom, the panels show proton density, bulk flow speed, proton temperature and magnetic field strength and components. The red dashed lines indicate the predicted window of CME arrival time from our ENLIL with Cone Model run (08:09–13:20 UT on 16 December 2008). We observed a magnetic cloud flux rope signature behind the front, highlighted by the blue dash-dotted lines. Full size image Since its launch, the dynamic twin viewpoints of STEREO have enabled studies of the true propagation of CMEs in 3D space. Our new elliptical tie-pointing technique uses the curvature of the CME front as a necessary third constraint on the two viewpoints to build an optimum 3D reconstruction of the front. Here, the technique is applied to an Earth-directed CME, to reveal numerous forces that take effect throughout its propagation. The early acceleration phase results from the rapid release of energy when the CME dynamics are dominated by outward magnetic and gas pressure forces. Different models can reproduce the early acceleration profiles of CME observations, although it is difficult to distinguish between them with absolute certainty [45] , [46] . For this event, the acceleration phase coincides with a strong angular expansion of the CME in the low corona, which tends towards a constant in the later observed propagation in the solar wind. Although, statistically, expansion of CMEs is a common occurrence [47] , it is difficult to accurately determine the magnitude and rate of expansion across the two-dimensional plane-of-sky images for individual events. Some studies of these single-viewpoint images of CMEs use characterizations such as the cone model [20] , [21] but assume the angular width to be constant (rigid cone), which is not always true early in the events [12] , [38] . Our 3D front reconstruction overcomes the difficulties in distinguishing expansion from image projection effects, and we show that early in this event there is a non-constant, power-law, angular expansion of the CME. Theoretical models of CME expansion generally reproduce constant radial expansion, based on the suspected magnetic and gas pressure gradients between the erupting flux rope and the ambient corona and solar wind [14] , [48] , [49] . To account for the angular expansion of the CME, a combination of internal overpressure relative to external gas and magnetic pressure dropoffs, along with convective evolution of the CME in the diverging solar wind geometry, must be considered [13] . During this early-phase evolution, the CME is deflected from a high-latitude source region into a non-radial trajectory, as indicated by the changing inclination angle ( Fig. 3b ). Although projection effects again hinder interpretations of CME position angles in single images, statistical studies show that, relative to their source region locations, CMEs have a tendency to deflect towards lower latitudes during solar minimum [39] , [50] . It has been suggested that this results from the guiding of CMEs towards the equator by either the magnetic fields emanating from polar coronal holes [8] , [9] or the flow pattern of the background coronal magnetic field and solar wind/streamer influences [19] , [51] . Other models show that the internal configuration of the erupting flux rope can have an important effect on its propagation through the corona. The orientation of the flux rope, either normal or inverse polarity, will determine where magnetic reconnection is more likely to occur, and therefore change the magnetic configuration of the system to guide the CME either equator- or poleward [10] . Alternatively, modelling the filament as a toroidal flux rope located above a midlatitude polarity inversion line results in non-radial motion and acceleration of the filament, because of the guiding action of the coronal magnetic field on the current motion [11] . Both these models have a dependence on the chosen background magnetic field configuration, and so the suspected drawn-out magnetic dipole field of the Sun by the solar wind [40] , [41] may be the dominant factor in deflecting the prominence/CME eruption into this observed non-radial trajectory. At larger distances from the Sun (>7 ), the effects of drag become important as the CME velocity approaches that of the solar wind. The interaction between the moving magnetic flux rope and the ambient solar wind has been suggested to have a key role in CME propagation at large distances at which the Lorentz driving force and the effects of gravity become negligible [4] . Comparisons of initial CME speeds and in situ detections of arrival times have shown that velocities converge on the solar wind speed [15] , [16] . For this event, we find that the drag force is indeed sufficient to accelerate the CME to the solar wind speed, and quantify that the kinematics are consistent with the quadratic regime of aerodynamic drag (turbulent, as opposed to viscous, effects dominate). The importance of drag becomes further apparent through the CME interaction with a slow-speed solar wind stream ahead of it, slowing it to a speed that accounts for the observed arrival time at L1 near Earth. This agrees with the conjecture that Sun–Earth transit time is more closely related to the solar wind speed than the initial CME speed [52] . Other kinematic studies of this CME through the HI fields of view quote velocities of 411 ± 23 km s −1 (Ahead) and 417 ± 15 km s −1 (Behind) when assumed to have zero acceleration during this late phase of propagation [34] , or an average of 363 ± 43 km s −1 when triangulated in time-elongation J-maps [36] . These speeds through the HI fields of view, lower than those quantified through the COR1/2 fields of view, agree somewhat with the deceleration of the CME to match the slow-speed solar wind ahead of it in our magnetohydrodynamic simulation. Ultimately, we are able to predict a more accurate arrival time of the CME front at L1. A cohesive physical picture for how the CME erupts, propagates and expands in the solar atmosphere remains to be fully developed and understood from a theoretical perspective. Realistic magnetohydrodynamic models of the Sun's global magnetic field and solar wind are required to explain all processes that take effect, along with a need for adequate models of the complex flux rope geometries within CMEs. In addition, ambitious space exploration missions, such as Solar Orbiter [53] (ESA) and Solar Probe+ [54] (NASA), will be required to give us a better understanding of the fundamental plasma processes responsible for driving CMEs and determining their adverse effects on Earth. CME front detection and characterization For the coronagraph images of COR1/2, a multiscale filter was used to determine a scale at which the signal-to-noise ratio of the CME was deemed optimal for the pixel-chaining algorithm to highlight the edges in the images [55] . To specifically determine the CME front, running and fixed difference masks were overlaid on the multiscale edge detections of both the Ahead and Behind viewpoints simultaneously, enabling us to confidently point and click along the relevant CME front edges in each image. For the Heliospheric images of HI1, a modified running difference was used to enhance the faint CME features by correcting for the apparent background stellar motion between frames [15] . The CME was scaled to an appropriate level for pointing and clicking along its front. Once the CME fronts were determined across each instrument plane of sky, an ellipse was fit to each front to characterize the changing morphology of the CME [38] . Elliptical tie pointing Three-dimensional information may be gleaned from two independent viewpoints of a feature using tie-pointing techniques to triangulate lines of sight in space [27] . However, when the object is known to be a curved surface, sight lines will be tangent to it and not necessarily intersect upon it. Consequently, CMEs cannot be reconstructed by tie pointing alone, but rather their localization may be constrained by intersecting sight lines tangent to the leading edges of a CME [56] , [57] . It is possible to extract the intersection of a given epipolar plane through the ellipse fits in both the Ahead and Behind images, resulting in a quadrilateral in 3D space. Inscribing an ellipse within the quadrilateral, such that it is tangent to all four sides [58] , [59] , provides a slice through the CME that matches the observations from each spacecraft. A full reconstruction is achieved by stacking ellipses from numerous epipolar slices. As the positions and curvatures of these inscribed ellipses are constrained by the characterized curvature of the CME front in the stereoscopic image pair, the modelled CME front is considered as an optimum reconstruction of the true CME front. This is repeated for every frame of the eruption to build the reconstruction as a function of time and view the changes to the CME front as it propagates in 3D. Following Horwitz [59] , we inscribe an ellipse within a quadrilateral using the following steps (see Fig. 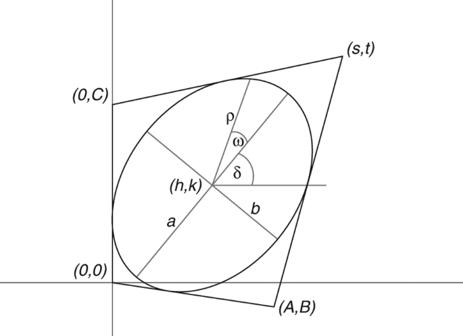Figure 5: An ellipse inscribed within a convex quadrilateral. An isometry of the plane is applied such that the quadrilateral has vertices (0,0), (A,B), (0,C), (s,t). The ellipse has a centre (h, k), a semimajor axisa, a semiminor axisb, a tilt angleδand is tangent to each side of the quadrilateral. 5 ): Figure 5: An ellipse inscribed within a convex quadrilateral. An isometry of the plane is applied such that the quadrilateral has vertices (0,0), ( A , B ), (0, C ), ( s , t ). The ellipse has a centre (h, k), a semimajor axis a , a semiminor axis b , a tilt angle δ and is tangent to each side of the quadrilateral. Full size image • Apply an isometry to the plane such that the quadrilateral has vertices (0, 0), ( A , B ), (0, C ), ( s , t ), where, in the case of an affine transformation, we set A =1, B =0 and C =1, with s and t as variables. • Set the ellipse centre point ( h , k ) by fixing h somewhere along the open line segment connecting the midpoints of the diagonals of the quadrilateral and hence determine k from the equation of a line, for example • To solve for the ellipse tangent to the four sides of the quadrilateral, we can solve for the ellipse tangent to the three sides of a triangle the vertices of which are the complex points and the two ellipse foci are then the zeroes of the equation the discriminant of which can be denoted by r ( h )= r 1 ( h )+ ir 2 ( h ) where Thus, we need to determine the quartic polynomial u ( h )=| r ( h )| 2 = r 1 ( h ) 2 + r 2 ( h ) 2 and we can then solve for the ellipse semimajor axis a and semiminor axis b from the equations by parameterizing R = a 2 − b 2 and W = a 2 b 2 to obtain • Knowing the axes, we can generate the ellipse and float its tilt angle δ until it sits tangent to each side of the quadrilateral, using the inclined ellipse equation where ω ′= ω + δ and ω is the angle from the semimajor axis to a radial line ρ on the ellipse. Drag modelling The evolution of CMEs as they propagate from the Sun through the heliosphere is a complex process, simplified by using a parameterized drag model. Comparing Equation (1) and Equation (2) where C D and M cme are approximately constant, and A cme and ρ sw are functions of distance expected to have a power-law form. We can therefore represent their combined behaviour as a single power law, as in Equation (12). For example, if we assume a density profile of ρ sw ( r )= ρ 0 r −2 , and a cylindrical CME of area A cme ( r )= A 0 r , then from Equation (12) we expect β =1. The α parameter, representative of the strength of the interaction, is then determined by the constants A 0 , M cme and C D , such that high-mass, small-volume CMEs are less affected by drag than are low-mass, large-volume CMEs. This method of parameterization has been shown to reproduce the kinematic profiles of a large number of events [44] . We assume an additional parameter γ to indicate the type of drag, suggested to be either linear ( γ =1) or quadratic ( γ =2). Although this parameterization may obscure some of the complex interplay between the various quantities, it does not affect the most crucial part that we are trying to test: Is aerodynamic drag an appropriate model and, if so, which regime (linear or quadratic) best characterizes the kinematics? A bootstrapping technique [60] was used to obtain statistically significant parameter ranges from the drag model of Equation (2). This technique involves the following steps: 1. An initial fit to the data y is obtained, yielding the model fit with parameters . 2. The residuals of the fit are calculated: . 3. The residuals are randomly resampled to yield ∈ *. 4. The model is then fit to a new data vector y *= y + ∈ * and the parameters are stored. 5. Steps 3–4 are repeated many times (10,000). 6. Confidence intervals on the parameters are determined from the resulting distributions. In our case, the model parameters were the initial height h cme of the CME at the start of the modelling; the speed v sw of the solar wind at 1 AU; the velocity v cme of the CME at the start of the modelling; and the drag parameters α , β and γ . To test for self-consistency, we allowed the observationally known parameters of initial CME height and velocity to vary in the bootstrapping procedure, and recovered comparable values. The parameters α and β were in reasonable agreement with values from previous studies [44] . How to cite this article: Byrne, J.P. et al . Propagation of an Earth-directed coronal mass ejection in three dimensions. Nat. Commun. 1:74 doi: 10.1038/ncomms1077 (2010).